Bactericidal activity of black silicon Black silicon is a synthetic nanomaterial that contains high aspect ratio nanoprotrusions on its surface, produced through a simple reactive-ion etching technique for use in photovoltaic applications. Surfaces with high aspect-ratio nanofeatures are also common in the natural world, for example, the wings of the dragonfly Diplacodes bipunctata . Here we show that the nanoprotrusions on the surfaces of both black silicon and D. bipunctata wings form hierarchical structures through the formation of clusters of adjacent nanoprotrusions. These structures generate a mechanical bactericidal effect, independent of chemical composition. Both surfaces are highly bactericidal against all tested Gram-negative and Gram-positive bacteria, and endospores, and exhibit estimated average killing rates of up to ~450,000 cells min −1 cm −2 . This represents the first reported physical bactericidal activity of black silicon or indeed for any hydrophilic surface. This biomimetic analogue represents an excellent prospect for the development of a new generation of mechano-responsive, antibacterial nanomaterials. Nanomaterials that possess topographical features with high aspect ratios frequently display remarkable surface properties, such as high hydrophobicity and strong biological activity on a cellular level [1] , [2] , [3] , [4] , [5] , [6] . The microbial contamination of surfaces remains a world wide research challenge. Recently we reported the wings of the cicada Psaltoda claripennis possessed potent bactericidal activity against Pseudomonas aeruginosa , an opportunistic human pathogen [7] , and showed their surfaces to be covered by an array of regularly spaced nanopillar structures. Furthermore, it was shown that the bactericidal nature of the cicada wing arose from physical phenomena based on the nanostructure of the surface, which appeared independent of the biochemical functionality of the wing [8] , [9] . On the basis of this underlying physical principle, other topologies that possess surface architectures which may exhibit similar structural characteristics were investigated. One such example is black silicon (bSi), which is a synthetic nanomaterial produced through a simple reactive-ion etching (RIE) technique to possess high aspect ratio nanoprotrusions. Black silicon was developed for photovoltaic and sensing applications [10] , [11] , [12] , [13] ; particularly for biomedical applications [14] , [15] , [16] , [17] . In this work, we investigate the antibacterial potential of the synthetic bSi surface, together with its related dragonfly Diplacodes bipunctata wing surface, and compare the antibacterial behaviour to that previously obtained for cicada wing surfaces. The physicochemical properties of bSi and native wing surfaces are chemically and structurally characterized prior to assessing their antibacterial activity against three different bacterial strains with a variety of cell wall structures. The surfaces of bSi and dragonfly are highly bactericidal against all tested Gram-negative and Gram-positive bacteria, and endospores, and both surfaces exhibit estimated average killing rates of up to ~450,000 cells min −1 cm −2 . This represents the first reported physical bactericidal activity of bSi or indeed for any hydrophilic surface. Surface nanoarchitecture Scanning electron microscopy (SEM) of the upper surface of bSi and dragonfly forewings ( Fig. 1a,b , Supplementary Fig. S1 ) showed disordered nanopillar systems having hierarchical topographical features that resulted from tip cluster formation through bending of the nanoprotrusions. Micrographs of surfaces tilted at an angle of 53° illustrated that the nanopillars of bSi are sharper and more distinct from one another, and approximately twice the height of those of the dragonfly wing. The dragonfly wing nanopillars tend towards a ‘network’ at their bases, whereas their tips remain disconnected or form tip clusters. These differences in microstructure are also seen in their respective optical profilometry images over broader areas (see Fig. 1c,d ), and in the three-dimensional (3D) reconstructions of the SEM images ( Fig. 1e,f , Supplementary Movie 1 ). 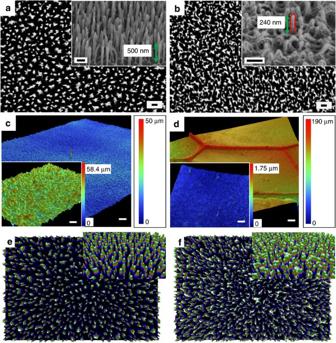Figure 1: Characterization of black silicon andD. bipunctatawings. Scanning electron micrographs of the upper surface of (a) bSi and (b) dragonfly forewings at × 35,000 magnification demonstrate the surface patterns of the two samples. Scale bars, 200 nm. Micrographs tilted at an angle of 53° (inset) show sharper nanopillars of black silicon distinct from one another and approximately twice the height of those of the dragonfly wing. Optical profilometry shows the nanoprotrusions of (c) bSi and (d) dragonfly forewings. Scale bars, 50 μm; inset, 2 μm. Three-dimensional reconstructions based on a displacement map technique further highlight the differences and similarities of (e) bSi and (f) dragonfly forewings. Figure 1: Characterization of black silicon and D. bipunctata wings. Scanning electron micrographs of the upper surface of ( a ) bSi and ( b ) dragonfly forewings at × 35,000 magnification demonstrate the surface patterns of the two samples. Scale bars, 200 nm. Micrographs tilted at an angle of 53° (inset) show sharper nanopillars of black silicon distinct from one another and approximately twice the height of those of the dragonfly wing. Optical profilometry shows the nanoprotrusions of ( c ) bSi and ( d ) dragonfly forewings. Scale bars, 50 μm; inset, 2 μm. Three-dimensional reconstructions based on a displacement map technique further highlight the differences and similarities of ( e ) bSi and ( f ) dragonfly forewings. Full size image The pillar characteristics, their spatial arrangement and nanopillar clusters present on the bSi and dragonfly were obtained using image analysis techniques (cicada wing surfaces were also used for comparison; Supplementary Fig. S2 ). Both the dragonfly wing and bSi surfaces clearly showed a random size, shape and spatial distribution of nano-clusters in their upper contact plane, whereas the cicada wing topology showed a regular array of pillars 50–70 nm in diameter, spaced ~200 nm apart, but containing 2D micro-domains due to stacking faults. Black silicon clusters spanned 20–80 nm diameters with a bimodal distribution, whereas dragonfly clusters showed a clear sigmoidal population distribution below 90 nm, with many of these clusters below 30 nm in diameter, which suggests the presence of a greater number of more complex, finer clusters. The spatial distributions of both bSi and dragonfly wing clusters ranged from 200 to 1,800 nm in diameter, which arises from the randomness in their perimeters. Clusters of bSi formed a broader spatial distribution than those present on the dragonfly wing surfaces. Tip cluster formation was more prevalent in the natural dragonfly wing surface due to the lower bending stiffness of the nanopillars, which depends upon shape, scale, respective Young’s moduli and material density [18] . Aizenberg and co-workers [19] have shown how capillary forces induce self-reorganization under the influence of the overall geometry and mechanical and surface properties. Such a secondary structure is also evident in the images derived from the 3D SEM reconstruction technique ( Fig. 1e,f ). X-ray photoelectron spectroscopy (XPS) analysis allowed the determination of the elemental composition of the top layers of the dragonfly wing and bSi surface. High-resolution scans (inset) were performed in ~20 eV intervals across the O 1 s and C 1 s peaks. Carbon to oxygen ratios ( Supplementary Fig. S3 ) indicated that the dragonfly surface was almost exclusively composed of longer chain hydrophobic lipids, whereas the bSi surface was primarily amorphous Si with a small degree of surface oxidation arising from the processing stage. Contact angle measurements indicated that the wing surfaces were superhydrophobic, whereas the bSi surfaces were relatively lower in hydrophobicity ( Table 1 ). Table 1 Feature comparison of insect wings and black silicon surfaces. Full size table Surface bactericidal activity To quantify the bactericidal properties of the bSi and the dragonfly wing surface, three species of bacteria were incubated on each surface for periods of up to 30 h and the bacterial viability monitored. The bacterial species examined represented the major prokaryotic taxa, and included Gram-negative P. aeruginosa ATCC 9027, Gram-positive Staphylococcus aureus 65.8 T , and both the vegetative cells and spores of Bacillus subtilis NCIMB 3610 T . The morphological appearance of all cells and spores that attached to the surface of the bSi and the dragonfly wings were found to be significantly different to those attaching to planar glass and silicon surfaces, which acted as control surfaces ( Fig. 2a–d, i–l ; controls given in Supplementary Fig. S4 ). The cellular integrity of all species appeared to be significantly disrupted by the nanopillars present on both of these substrata despite the significant difference in surface chemistry and hydrophobicity ( Fig. 2 and Supplementary Fig. S4 ). Significant deformation and engulfment can be seen with not only the three vegetative cell types but also with B. subtilis spores. We previously observed similar physical deformations of P. aeruginosa cells that attached to cicada wings, which were subsequently found to be inactivated after attachment. A viability analysis of the cells in contact with the bSi and dragonfly wings using confocal laser scanning microscopy confirmed that all cells and spores were also non-viable after attachment ( Fig. 2e–h,m–p ). Cell disruption was assessed using the fluorescent dye propidium iodide which penetrates all ruptured cells, causing red fluorescence, indicating inactivation. Notably, the bSi and dragonfly wing surfaces were effective not only against the Gram-negative P. aeruginosa cells but also against Gram-positive S. aureus and B. subtilis cells. The cicada wing studies previously performed highlighted that the cicada wing substrata were effective only against the Gram-negative cells [7] . Gram-positive cells are generally more rigid and more resistant to mechanical lysis than Gram-negative cells due to their peptidoglycan cell wall being ~4–5 times thicker than those of the Gram-negative bacteria [20] . This greater cell wall thickness requires a greater deformational stress to disrupt the cell wall, deform the inner membrane and cause cell death. In addition to being effective against vegetative bacterial cells examined, the bSi and dragonfly surface nanoarchitectures were clearly able to disrupt the multilayer spore coat, which controls the viability of the spores [21] , [22] . The spore coating affords great durability and resistance against external stresses such as desiccation, making spores the most effective means of bacterial survival under stress conditions. The results obtained in this study indicated that the deforming stress applied by both bSi and D. bipunctata wings to the bacterial cells is substantial, and demonstrated the significant potential for bSi topologies to be used in counteracting bacterial survival strategies. The interaction between the Gram-negative bacteria and the cicada wing nanopillars, leading to bactericidal activity, was previously shown to be dependent on the physical structure of the surface and cell rigidity, as recently demonstrated by the application of microwave irradiation to cells with rigid wall structures [7] , [8] , [9] . The nano-mechanical basis of the bactericidal effect was further confirmed by sputter-coating the bSi and dragonfly wing surfaces with gold. The gold modified surfaces also displayed activity against cells and spores ( Supplementary Fig. S5 ), which is consistent with the data previously reported for gold-coated cicada wing surfaces, which exhibited activity against Gram-negative bacteria [7] , [8] . 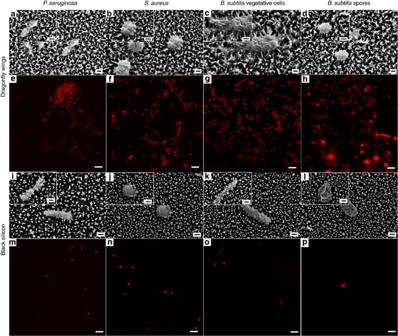Figure 2: Cell morphology on dragonfly wings and black silicon. SEM images ofP. aeruginosa,S. aureus,B. subtilisvegetative cells andB. subtilisspores appear to be significantly disrupted through interaction with both the dragonfly wing (a–d) and bSi (i–l). Scale bars, 200 nm. Confocal laser scanning micrographs confirm that disruption by dragonfly wing (e–h) and bSi (m–p) was lethal to the cells; non-viable bacterial cells and spores were stained with propidium iodide (red), whereas the living cells were stained with SYTO 9 (green). All cells appeared red, indicating the high efficiency of surfaces in inactivating the bacteria. Scale bars, 5 μm. Figure 2: Cell morphology on dragonfly wings and black silicon. SEM images of P. aeruginosa , S. aureus , B. subtilis vegetative cells and B. subtilis spores appear to be significantly disrupted through interaction with both the dragonfly wing ( a – d ) and bSi ( i – l ). Scale bars, 200 nm. Confocal laser scanning micrographs confirm that disruption by dragonfly wing ( e – h ) and bSi ( m – p ) was lethal to the cells; non-viable bacterial cells and spores were stained with propidium iodide (red), whereas the living cells were stained with SYTO 9 (green). All cells appeared red, indicating the high efficiency of surfaces in inactivating the bacteria. Scale bars, 5 μm. Full size image Bactericidal efficiency The bactericidal efficiency of the bSi and the D. bipunctata wing surfaces was quantitatively assessed over periods up to 30 h using a standard viability plate-count technique. This plate-count assay was adopted according to the FDA protocols for the evaluation of foodstuff sterilization, with an adjustment made to the inoculum size to accommodate an evaluation of the antibacterial potential of surfaces rather than that of a bulk sterilization technique [23] . The number of colony forming units in suspensions of all cell types tested were shown to significantly decrease over 30 h incubation ( Fig. 3 ). On the basis of these numbers, the killing efficiency of the bSi surface and dragonfly wings over the first 3 h against the four cell types tested were quantified ( Fig. 4 ). The number of cells killed by the bSi and the dragonfly wings was determined as the difference between the number of surviving cells and those remaining in the control after the same incubation period, in order to account for the low levels of natural cell death that occurs in low-nutrient conditions. The bactericidal activities of these topologically related surfaces appeared to be largely comparable; both surfaces had killing rates of ~450,000 cells min −1 cm −2 over the first 3 h which then declined to ~50,000 cells min −1 cm −2 for S. aureus . When this killing efficiency is compared with the number of cell of each type required to infect an individual, that is, the minimum infective dose ( P. aeruginosa – 10 3 cells, S. aureus – 10 5 cells, and Bacillus cereus as a representative of the non-pathogenic B. subtilis – 10 5 cells) [24] , [25] , [26] , it becomes clear that these samples would be highly effective antibacterial surfaces. For example, a sample of bSi 1 cm 2 in size would be capable of killing the minimum infective dose of S. aureus cells 810 times over 3 h, and in the case of P. aeruginosa this increases to 77,400 times the minimum infective dose. Analysis of the bactericidal activities in direct experiments with bSi surfaces in nutrient rich environments has indicated that viable cells in the infective dose range were eliminated after 6 h ( Supplementary Methods and Supplementary Fig. S6 ). 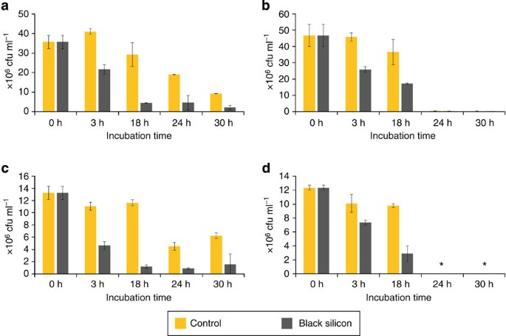Figure 3: Bactericidal activity of black silicon surfaces. Counts of viable cells of (a)P. aeruginosa, (b)S. aureus, (c)B. subtilisand (d)B. subtilisspores remaining in suspension when incubated with bSi and control suspensions for up to 30 h. At longer time intervals (24 and 30 h) cell numbers tended to also decrease in the controls due to the nutrient-poor medium. Data for spores in suspension after 24 and 30 h are not available due to the germination of spores after 18 h. Error bars are s.d. values. Figure 3: Bactericidal activity of black silicon surfaces. Counts of viable cells of ( a ) P. aeruginosa , ( b ) S. aureus , ( c ) B. subtilis and ( d ) B. subtilis spores remaining in suspension when incubated with bSi and control suspensions for up to 30 h. At longer time intervals (24 and 30 h) cell numbers tended to also decrease in the controls due to the nutrient-poor medium. Data for spores in suspension after 24 and 30 h are not available due to the germination of spores after 18 h. Error bars are s.d. values. 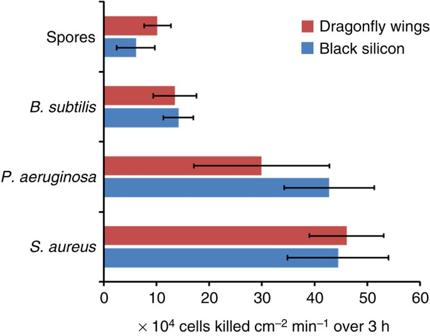Figure 4: Bactericidal efficiency of black silicon and dragonfly wings. The bactericidal efficiency of both the bSi andD. bipunctatawing surfaces over the first 3 h of incubation was calculated as the number of cells killed per square centimetre of projected sample surface area, per minute of incubation time. The number of cells killed was determined by subtracting the number of surviving cells from the number of cells remaining in controls at the corresponding time interval. The uncertainty values represent the natural variability associated with biological systems, and were calculated based on standard deviations in colony forming units. Error bars are based on s.d. values. Full size image Figure 4: Bactericidal efficiency of black silicon and dragonfly wings. The bactericidal efficiency of both the bSi and D. bipunctata wing surfaces over the first 3 h of incubation was calculated as the number of cells killed per square centimetre of projected sample surface area, per minute of incubation time. The number of cells killed was determined by subtracting the number of surviving cells from the number of cells remaining in controls at the corresponding time interval. The uncertainty values represent the natural variability associated with biological systems, and were calculated based on standard deviations in colony forming units. Error bars are based on s.d. values. Full size image There have been recent advances in both direct AFM measurement of bacterial cells, particularly with a view to examining the mechanical properties of cell walls and their internal osmotic turgor pressures [27] , [28] . For example, applying both modelling and direct AFM measurements, Deng et al. [29] quantified the cell wall Young’s moduli of live E. coli as 23 and 49 MPa for axial and circumferential directions, whereas the cell turgor pressure was 29 kPa, through the analysis of the cell bulging strain under an externally imposed perturbation. As a consequence of the wall tension brought about by the indenting deformation, significant power law stress stiffening of peptidoglycan network of the cell wall was seen to have an exponent 1.2. Here, we see that the competition between the elasticity of the cell membrane and the capillarity of the bSi and dragonfly wing architecture compared to cicada surfaces favors enhanced engulfment with its increased deformation and cell wall stress [7] , which is further increased with the longer, more pronounced nanospikes of the bSi ( Supplementary Methods and Supplementary Fig. S7 ). The extensive bactericidal activity displayed by the synthetic bSi provides an opportunity for a new approach to mechano-responsive microbiology, whereby the cell responds to the physical interaction forces of the surface structures (and their accompanying stresses), leading to cell deformation and death. The ability to readily fabricate such nanomaterials suggests their potential for use in the development of a wide range of bactericidal surfaces for use in biomedical and industrial applications. Our results demonstrated that (i) the nanostructured bSi and the natural D. bipunctata dragonfly wings are highly effective bactericidal surfaces, with the bactericidal activity being driven by mechanical and structural responses to the deformational stresses imposed by the surface nanoarchitecture on the peptidoglycan cell wall and inner membrane of bacterial cells, (ii) synthetic antibacterial nanomaterials that exhibit a similar effectiveness to the dragonfly wing surface structures in killing bacterial cells can be readily fabricated over large areas. These surfaces appear to be effective, independent of their surface chemical functionality, and (iii) such synthetic surfaces exhibit a bactericidal activity that is comparable to their natural counterparts and this may be further enhanced via optimization. These data provide a clear demonstration of the impact that mechano-responsive surfaces could play in countering microbial contamination, suggesting that novel antimicrobial nanomaterials may open the way for new applications in the field of mechano-microbiology. Reactive-ion beam etching Black silicon was produced via RIE as described elsewhere [30] , [31] , [32] , [33] . RIE with SF 6 and O 2 was performed for 5 min to produce the nanopillars on silicon wafers using an Oxford PlasmaLab 100 ICP380 instrument. A p-type boron-doped 100 mm-diameter commercial Si wafer with specific resistivity of 10–20 Ω cm −1 , (100) oriented surface and 525±25 μm thickness (Atecom Ltd, Taiwan) was used as a substrate for the bSi formation. Separation between pillars was proportional to the etching time as ∝ t 0.5 . Insect wing preparation Dragonfly specimens ( D. bipunctata , Order Odonata ) were collected from the Brisbane (Australia) parkland areas. The wings were precisely dissected using either scissors or a scalpel. These were then attached to circular discs by double sided adhesive tapes, then rinsed with copious quantities of MilliQ water (resistivity of 18.2 MΩ cm −1 , Millipore, Billerica, MA, USA) followed by drying with 99.99% purity nitrogen gas. Characterization of surface nanoarchitecture High-resolution electron micrographs of bSi and dragonfly wings were recorded using a field-emission SEM (FESEM; ZEISS SUPRA 40 VP, Oberkochen, BW, Germany) at 3 kV under × 35,000, × 70,000, × 150,000 and × 1,000,000 magnification. Prior to viewing, the wing samples were coated with thin gold films using a Dynavac CS300 (ref. 34 ). Several fields of view were recorded, including various sections of bSi samples and multiple regions of the wings, to confirm morphological consistency. The surface architecture was analysed initially using a Bruker AXS Contour GT 3D optical profiling system in white light vertical scanning interferometry mode using × 4, and × 230 objective lenses. Three samples were scanned to evaluate the overall homogeneity of the surface, prior to detailed topographical profiles at five different locations on the surface. As the feature size of the nanostructures on bSi and the wing surfaces was below the optical resolution limit, their architecture was observed from the noise pattern of the optical images. Characterization of surface chemical compositions XPS was performed using a Kratos Axis Ultra DLD X-ray photoelectron spectrometer (Kratos Analytical Ltd., UK) equipped with a monochromatic X-ray source (Al Kα, hυ =1486.6 eV) operating at 150 W. The spectrometer energy scale was calibrated using the Au 4f 7/2 photoelectron peak at binding energy of 83.98 eV. Samples were flooded with low-energy electrons during the analysis to counteract surface charging. The hydrocarbon component of the C 1 s peak (binding energy 285.0 eV) was used as a reference for charge correction. The elements present on the surfaces were determined from survey spectra in the range 0–1400, eV at an interval and pass energy of 1 and 160 eV, respectively. The relative atomic concentration of elements detected by XPS was quantified on the basis of the peak area in the survey spectra using sensitivity factors for the Kratos instrument. High-resolution scans were performed across each of the C 1 s, O 1 s and Si 2p peaks, which were then fitted with Gaussian–Lorentzian components after the removal of a linear background signal (Kratos Vision II software). Image analysis was carried out with Image J software (Ver. 1.47, Wayne Rasband, National Institute of Health, USA). Surface wettability Static water contact angles were measured on bSi and the wing using the sessile drop method [7] . The contact angle measurements were carried out in air using an FTA1000c equipped with a nanodispenser (First Ten Ångstroms, Inc., Portsmouth, VA, USA). Volumes of the droplets were ~1.0 μl. The contact angles were measured by recording 50 images over 2 s with a Pelco model PCHM 575-4 camera and measuring contact angles after the droplet had rested on the surface for ~1 s. Bacterial growth conditions and sample preparation Three strains were used: P. aeruginosa ATCC 9027, Staphylococcus aureus CIP 65.8 T and Bacillus subtilis NCIMB 3610 T . The selected strains are typical representatives of three large bacterial taxonomic lineages and were obtained from American Type Culture Collection (ATCC, Manassas, VA, USA), Culture Collection of the Institute Pasteur (CIP, Paris, France) and the National Collection of Industrial, Food and Marine Bacteria (NCIMB, Aberdeen, UK). Prior to each bacterial attachment experiment, bacterial cultures were refreshed on nutrient agar from stocks (Oxoid, Basingstoke, Hampshire, UK). Fresh bacterial suspensions were grown overnight at 37 °C in 5 ml of nutrient broth (Oxoid, Basingstoke, Hampshire, UK). Bacterial cells were collected at the logarithmic stage of growth and the suspensions were adjusted to OD 600 =0.3. The insect wings, mounted on circular discs, were immersed in 5 ml of the bacterial suspension for incubation intervals of either 1, 3 or 18 h. For spore formation, an aliquot from the vegetative cell suspension of B. subtilis NCIMB 3610 T was spread on to the nutrient agar (Oxoid) plate and incubated at 37 °C for 7 days in depletion of oxygen. Sporulation (>95%) was observed microscopically on glass slides by staining spores with malachite green and counter-staining healthy cells with safranin [35] . Spores were then suspended in phosphate buffered saline (PBS) solution, washed at 13,000 r.p.m. for 5 min and re-suspended. Before incubation on the insect wings, the spore suspension in PBS was adjusted to OD 600 =1. The insect wings were then incubated with spore suspension for 1, 3 and 18 h attachment experiments. Cell viability analysis Confocal laser scanning microscopy was used to visualize the proportions of live cells and dead cells using LIVE/DEAD BacLight Bacterial Viability Kit, L7012. A mixture of SYTO 9 and propidium iodide fluorescent dyes (Molecular Probes, Invitrogen, Grand Island, NY, USA). SYTO 9 permeated both intact and damaged membranes of the cells, binding to nucleic acids and fluorescing green when excited by a 485 nm wavelength laser. On the other hand, propidium iodide alone entered only cells with significant membrane damage, which are considered to be non-viable, and binds with higher affinity to nucleic acids than SYTO 9. Bacterial suspensions were stained according to the manufacturer’s protocol, and imaged using a Fluoview FV10i inverted microscope (Olympus, Tokyo, Japan). For spore staining, a minor modification was made to this protocol [36] . Spores were stained with a mixture of 0.9 mmol l −1 of propidium iodide and 5 μmol l −1 of SYTO 9 for 15–20 min. The samples were then imaged under the confocal microscope. Bacterial viability plate counts Viability assays were performed by standard plate counts [37] . P. aeruginosa, S. aureus and B. subtilis cells and spores were suspended in 5 ml of PBS and adjusted to OD 600 =0.1. Re-suspended cells were diluted 1:10; then incubated in 3.5 cm diameter wells in triplicate with each well containing a 1 cm 2 area substratum sample of either a D. bipunctata wing, bSi, smooth silicon wafer or a glass cover slip. The cell suspensions were then sampled (100 μl) at discrete time intervals (3 and 18 h), serially diluted 1:10, and each dilution spread on three nutrient agar plates. Resulting colonies were then counted, and the number of colony forming units per mL was calculated. The number of colony forming units was assumed to be equivalent to the number of live cells in suspension [37] . The maximum bactericidal efficiency was measured as the number of inactivated cells per square centimetre of sample per minute of incubation time, calculated by subtracting the number of cells remaining in suspension from the corresponding control conditions. How to cite this article: Ivanova, E. P. et al. Bactericidal activity of black silicon. Nat. Commun. 4:2838 doi: 10.1038/ncomms3838 (2013).